Target control of complex networks Controlling large natural and technological networks is an outstanding challenge. It is typically neither feasible nor necessary to control the entire network, prompting us to explore target control: the efficient control of a preselected subset of nodes. We show that the structural controllability approach used for full control overestimates the minimum number of driver nodes needed for target control. Here we develop an alternate ‘ k -walk’ theory for directed tree networks, and we rigorously prove that one node can control a set of target nodes if the path length to each target node is unique. For more general cases, we develop a greedy algorithm to approximate the minimum set of driver nodes sufficient for target control. We find that degree heterogeneous networks are target controllable with higher efficiency than homogeneous networks and that the structure of many real-world networks are suitable for efficient target control. In the past decade network science offered deep insights into the structure and dynamics of complex networked systems [1] , [2] , [3] , [4] , [5] , [6] , [7] . Yet, we continue to lack tools to efficiently control the dynamics of complex networks. According to control theory [8] , [9] , [10] , a dynamic system is controllable if suitable external inputs can move the internal state of the system from any initial state to an arbitrary accessible final state in a finite time interval [11] . Recently, we introduced an analytical framework to study the controllability of complex networks via a combination of tools from network science, control theory and statistical physics [12] . By mapping the structural controllability problem [13] to a maximum matching problem [14] , we were able to identify a minimum set of driver nodes of size N D , sufficient to control the whole network [12] , [15] . For engineered systems, such as the auto-pilot system of an airplane, full control is essential. However, many biological, technological and social systems are massive in size and complexity, hence it is neither feasible nor necessary to control the full network. Instead, it is more realistic and sufficient to achieve target control, that is, to control a subset of target nodes (or a subsystem) that are essential for the system’s mission pertaining to a selected task. While potential applications of target control have been developed in domain-specific areas in biology [16] , chemical engineering [17] , epidemics [18] and economic networks [19] , a principled approach to identify a minimum set of driver nodes sufficient for the targeted control of an arbitrary complex network remains an open problem. We study two distinct schemes for choosing the subset of nodes we wish to control. In the random scheme, a fraction f of nodes are chosen uniformly at random. In the local scheme, the chosen nodes form a connected component, capturing a well-defined local network neighbourhood. To develop an efficiency measure of target control, we compare P D , which is the minimum number of driver nodes needed to control the fraction f of target nodes, with fN D , which is the corresponding relative fraction of the driver nodes needed for full control. If P D is less than fN D then target control is more efficient than full control for a given f . We also establish the overall target control efficiency by considering the integrated efficiency across the entire range of 0< f ≤1. For both scale-free (SF) [20] and Erdös–Rényi (ER) networks [21] , [22] , we find that in general, local target control is more efficient than random target control. More surprisingly, we find that degree heterogeneous networks, such as SF networks, have higher specific and overall target control efficiency than degree homogeneous networks, for both random and local schemes, when the average degree of the network is large. In contrast, for full control, degree homogeneous networks, such as ER networks, are more efficient than the corresponding degree heterogeneous networks [12] . Finally, we apply our methods to real data, confirming that many real-world networks display high efficiency of target control. Model The dynamics of most real systems is driven by nonlinear processes. However, the dynamical rules of real-world networks are so diverse that writing a general dynamical equation that captures them all is plainly impossible. Moreover, for many networks, especially biological networks, we do not even know the dynamical rules. Thus, before we explore the fully nonlinear dynamical problem, we have to understand the impact of the topological characteristics on linear control, which naturally serves as a prerequisite of the nonlinear controllability problem. Furthermore, the controllability of nonlinear systems is often structurally similar to and determined by the system’s linearized dynamics [23] . Indeed, a basic starting point for exploring the controllability of any nonlinear system is the study of the linearized version of the nonlinear dynamical system. Therefore, we start with the canonical linear time-invariant dynamics. where , and represent the system’s state, input and output vector, respectively. , and denote the state, input and output matrices, respectively. A captures the wiring diagram of the system; B identifies the nodes that are controlled by an external controller and u is the time-dependent input applied to the nodes in B ; C is the output matrix identifying the target nodes we want to control. For a network with node set , we are interested in controlling a target node set of size . We set the output matrix C =[ I ( c 1 ), I ( c 2 ),... I ( c S )], where I ( i ) denotes the i th row of an N × N identity matrix I . The system ( A , B , C ) is said to be target controllable with respect to a given target node set C if there exists a time-dependent input vector u ( t )=( u 1 ( t ),... u M ( t )) T that can drive the state of the target nodes to any desired final state in finite time. Target controllability can be viewed as a special type of output controllability and the system ( A , B , C ) is target controllable if and only if the dimension of the output controllable subspace d ( A , B , C ) satisfies representing the mathematical condition for target controllability [24] . Note that when S = N , C is the identity matrix and (2) reduces to the Kalman condition for full controllability [11] . If (2) is satisfied, for initial condition x (0)=0, we can compute the optimal input vector u ( t ) such that we can reach the desired final state with minimum energy cost in time (that is, ) (ref. 24 ). where ( Supplementary Note 1 ). In some ways the target control problem is more difficult than the full control problem. Full control has a graphical condition, which can be easily checked by exactly mapping the controllability problem to the maximum matching problem. Target control lacks such an exact mapping. Therefore, to solve the target control problem in the single-input case, we develop a new approach that we call the ‘ k -walk theory’ ( Fig. 1 ; Supplementary Fig. 1 ; Supplementary Note 2 ). This theory is based on the principle that a node can control a target set of nodes provided that the length of the path from the control node to each target node in the set is unique. Using the k -walk theory, we can identify all sets of nodes that can be controlled by the given node. We show that the k -walk theory is more powerful than the standard approach as it can find controllable subsystems that the structural control theory misses ( Fig. 1 ; Supplementary Note 2 ). We rigorously prove that the k -walk theory is correct for directed tree-like networks, that is, networks with no loops ( Supplementary Note 2 ). 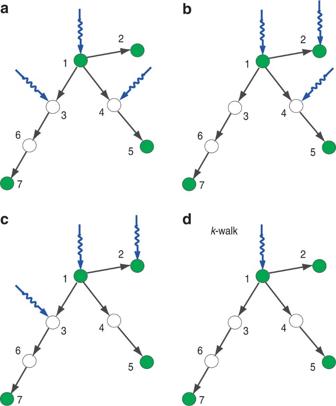Figure 1: Structural control theory versus thek-walk theory for target control. To control the whole network, the structural control theory predicts that we need at least three driver nodes. The possible choices for the sets of driver nodes are shown ina–c. If instead we want to control a subset of nodes, for example, {1, 2, 5, 7} (green nodes) with a minimum set of nodes, we need to solve the target control problem. The upper bound obtained by structural control theory indicates that we need at least three driver nodes (the same sets are shown ina,bandc). (d) But, in reality, we only need one driver node (node 1), which can be obtained from both thek-walk theory and the greedy algorithm, because the length of the path from the node 1 to each target node {1, 2, 5, 7} is unique. Figure 1: Structural control theory versus the k -walk theory for target control. To control the whole network, the structural control theory predicts that we need at least three driver nodes. The possible choices for the sets of driver nodes are shown in a – c . If instead we want to control a subset of nodes, for example, {1, 2, 5, 7} (green nodes) with a minimum set of nodes, we need to solve the target control problem. The upper bound obtained by structural control theory indicates that we need at least three driver nodes (the same sets are shown in a , b and c ). ( d ) But, in reality, we only need one driver node (node 1), which can be obtained from both the k -walk theory and the greedy algorithm, because the length of the path from the node 1 to each target node {1, 2, 5, 7} is unique. Full size image Although powerful, the k -walk theory is only applicable for the single-input case. For networks that require >1 control input, we formulate the target control problem in graph theoretic terms, allowing us to develop a greedy algorithm (GA) that offers a good approximation to the minimum set of inputs sufficient for target control ( Fig. 2 ). We rigorously prove that the input set selected by our algorithm can indeed control all target nodes ( Fig. 3 ; Supplementary Note 3 ). Both the k -walk theory and the GA are based on the structural control theory, that is, the system parameters are either fixed at zero or are independent free parameters. This approach has lead to several recent advances on network control [19] , [25] , [26] , [27] , [28] , [29] , [30] , [31] , [32] , [33] , [34] . Structural control theory, in general, relies on the canonical linear time-invariant dynamics of the system as discussed in the Methods. 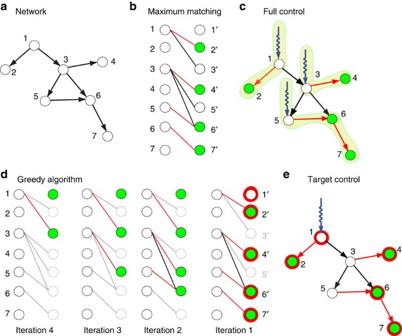Figure 2: Controlling a small network. (a) A directed network with seven nodes. (b) Maximum matching of the network in its bipartite representation. Matching edges are shown in red, matched nodes {x2,x4,x6,x7} are green and unmatched nodes {x1,x3,x5} are white. (c) By controlling the three unmatched nodes (driver nodes) and ensuring that there are no inaccessible nodes, the system is guaranteed to be structurally controllable. The underlying control skeleton (or the cactus structure) is highlighted. (d) Greedy algorithm developed for target control. Here the target set is {x1,x2,x4,x6,x7} (highlighted in red). In the first iteration, we match all target nodes by solving a maximum matching problem on an induced bipartite graph. Target nodes {x2,x4,x6,x7} (in green) are matched by {x1,x3,x5,x6}, which are the new target nodes considered in iteration 2. After four iterations, we obtain that nodex1is the driver node for the target set {x1,x2,x4,x6,x7}. (e) By controlling the unmatched nodex1calculated from the GA, the target set {x1,x2,x4,x6,x7} is guaranteed to be controllable. The red lines are the matched links obtained in the first iteration of greedy algorithm. This can be proved by interpreting GA as a backtracking process on the dynamic graph representation of the system (Supplementary Note 3). The upper bound ofPDcan be calculated by the minimal number of disjoint cacti that cover all target nodes, that is,for the target nodes {1, 2, 4, 6, 7}. The lower bound ofPDis just given by the first iteration of the greedy algorithm, that is,for the target nodes {1, 2, 4, 6, 7}, because in the first iteration only node 1 is unmatched. Figure 2: Controlling a small network. ( a ) A directed network with seven nodes. ( b ) Maximum matching of the network in its bipartite representation. Matching edges are shown in red, matched nodes { x 2 , x 4 , x 6 , x 7 } are green and unmatched nodes { x 1 , x 3 , x 5 } are white. ( c ) By controlling the three unmatched nodes (driver nodes) and ensuring that there are no inaccessible nodes, the system is guaranteed to be structurally controllable. The underlying control skeleton (or the cactus structure) is highlighted. ( d ) Greedy algorithm developed for target control. Here the target set is { x 1 , x 2 , x 4 , x 6 , x 7 } (highlighted in red). In the first iteration, we match all target nodes by solving a maximum matching problem on an induced bipartite graph. Target nodes { x 2 , x 4 , x 6 , x 7 } (in green) are matched by { x 1 , x 3 , x 5 , x 6 }, which are the new target nodes considered in iteration 2. After four iterations, we obtain that node x 1 is the driver node for the target set { x 1 , x 2 , x 4 , x 6 , x 7 }. ( e ) By controlling the unmatched node x 1 calculated from the GA, the target set { x 1 , x 2 , x 4 , x 6 , x 7 } is guaranteed to be controllable. The red lines are the matched links obtained in the first iteration of greedy algorithm. This can be proved by interpreting GA as a backtracking process on the dynamic graph representation of the system ( Supplementary Note 3 ). The upper bound of P D can be calculated by the minimal number of disjoint cacti that cover all target nodes, that is, for the target nodes {1, 2, 4, 6, 7}. The lower bound of P D is just given by the first iteration of the greedy algorithm, that is, for the target nodes {1, 2, 4, 6, 7}, because in the first iteration only node 1 is unmatched. 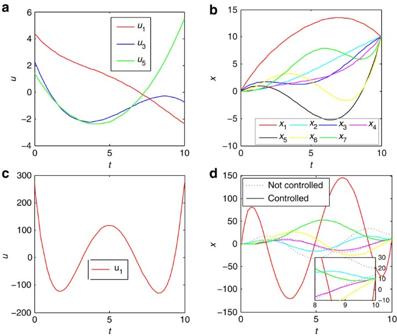Figure 3: Full versus target control of the simple network shown inFig. 1. (a,b) Full control. (a) The time-dependent input signalsu1(t),u3(t) andu5(t) predicted by equation (3) that can drive the state of the network from the initial state (x1=...=x7=0) to the final state (x1=...=x7=10). (b) The state trajectories of all nodes from initial state to the desired final state. (c,d) Target control. (c) The input required for the driver node 1 to control the state of the target nodes {1, 2, 4, 6, 7} from the initial state (x1=...=x7=0) to the final state (x1=x2=x4=x6=x7=10). (d) The state trajectories of all nodes fortε[0, 10], where the target nodes go from 0 to the desired state 10 (solid curves) and the uncontrolled nodes go from 0 to other values (dotted curves) whent=10. The inset indshows the detail of the final state of all seven nodes, which clearly shows that all the target nodes are controlled to be 10 and other uncontrolled nodes are not 10 and with finite values. Full size image Figure 3: Full versus target control of the simple network shown in Fig. 1 . ( a , b ) Full control. ( a ) The time-dependent input signals u 1 ( t ), u 3 ( t ) and u 5 ( t ) predicted by equation (3) that can drive the state of the network from the initial state ( x 1 =...= x 7 =0) to the final state ( x 1 =...= x 7 =10). ( b ) The state trajectories of all nodes from initial state to the desired final state. ( c , d ) Target control. ( c ) The input required for the driver node 1 to control the state of the target nodes {1, 2, 4, 6, 7} from the initial state ( x 1 =...= x 7 =0) to the final state ( x 1 = x 2 = x 4 = x 6 = x 7 =10). ( d ) The state trajectories of all nodes for t ε[0, 10], where the target nodes go from 0 to the desired state 10 (solid curves) and the uncontrolled nodes go from 0 to other values (dotted curves) when t =10. The inset in d shows the detail of the final state of all seven nodes, which clearly shows that all the target nodes are controlled to be 10 and other uncontrolled nodes are not 10 and with finite values. Full size image Previous studies based on the structural control theory shed some light on how to determine the upper bound of the minimum number of driver nodes for target controllability [35] , [36] . We can use the maximum matching method to find the minimum set of driver nodes ( N D nodes) for full control of the network ( Fig. 2a–c ). This results in N D disjoint ‘cacti’ ( Supplementary Note 3 ), each denoting the control region of a particular driver node under one specific maximum matching. We can then count the minimal number of disjoint cacti that cover all target nodes, which yields an upper bound of P D for target control (denoted as ) (see Fig. 2 ; Supplementary Note 3 for details). The lower bound of P D , denoted with , can also be obtained using maximum matching. We consider the maximum matching in a bipartite graph connecting on one side (1) the target nodes ( nodes), and on the other (2) the nodes that can reach the target nodes via (3) the edges among them. If a target node is unmatched, we must drive it directly, and the number of unmatched target nodes is the lower bound of P D . Taking Fig. 2 for example, the lower bound of P D is given by the first iteration of the GA, that is, for the target nodes {1, 2, 4, 6, 7}, because in the first iteration only node 1 is unmatched. Target controllability To quantify the efficiency of target control for a specific fraction f , we define the target controllability parameter α D ≡ P D / N D (Methods section) and investigate it for both random and local control schemes, as shown in Fig. 4a,d , respectively. Note that for f =1, we have α D =1 as target control reduces to full control. In Fig. 4 the black lines denote the neutral condition ( α D = f ) and serve as a benchmark because they mean that controlling an f fraction of target nodes requires an f fraction of the driver nodes needed for full control, that is, P D = fN D . In each figure, UB denotes the upper bound of the minimum number of driver nodes needed to control an f fraction of target nodes, predicted by the structural control theory ( Supplementary Note 3 ). Likewise, GA denotes the results of the greedy algorithm and LB ( Supplementary Note 3 ) denotes the lower bound, which is obtained by the first step of the GA (Methods section). 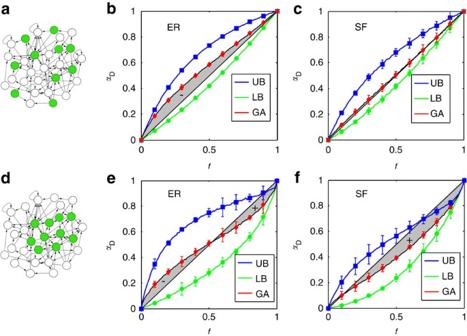Figure 4: Random versus local target controllability of two canonical network models. (a–c) Random selection scheme. (a) Illustrating random selection off=1/3 target nodes. (b) For ER networks with average degree ‹k›=5.6, we show the normalized fraction of driver nodes (αD) in function of the target node fractionffor the random selection scheme. (c) For SF networks with ‹k›=5.6 and exponentγ=2.4, we show the normalized fraction of driver nodes (αD) as a function of the target node fractionffor the random scheme. (d–f) Local selection scheme. (d) The selection of anf=1/3 target node with the local scheme. (e) For ER networks with the same average degree as inb, we show the normalized fraction of driver nodes (αD) in function of the target node fractionffor the local scheme. (f) For SF networks with the same ‹k› andγas inc, we show the normalized fraction of driver nodes (αD) as a function of the target node fractionffor the local scheme. The black line describes the neutral case, that is,αD=f(orPD=fND) when the target control has the same efficiency as the full control. In each figure, we denote UB as the upper bound, GA as the greedy algorithm and LB as the lower bound of the minimum number of driver nodes to control anffraction of target nodes. For ER networks, random target control is always less efficient than the full control, and for local target control efficiency depends onf. For SF networks random target control is as efficient as full control, but significant gains in efficiency are observed for local target control. Furthermore, for ER and SF networks local target control is more efficient than random target control. All results are averaged over 200 independent realizations of the networks with 104nodes. Figure 4b shows the results of random target control of ER networks. Here the GA curve is above the neutral line ( α D > f ), which indicates that the target control is less efficient than the neutral expectation. Figure 4c shows the results of random target control on SF networks and the GA curve is almost at the neutral line ( α D ≈ f ), which indicates that target control is as efficient as the neutral expectation. If we apply the local target control scheme to an ER network, we observe reduced efficiency for f <0.5 (minus symbol in Fig. 4e ) and enhanced efficiency for f >0.5 (plus symbol in Fig. 4e ). Figure 4f shows the case of local target control on SF networks, charactering that the target control is more efficient (that is, α D < f ). Figure 4: Random versus local target controllability of two canonical network models. ( a – c ) Random selection scheme. ( a ) Illustrating random selection of f =1/3 target nodes. ( b ) For ER networks with average degree ‹ k ›=5.6, we show the normalized fraction of driver nodes ( α D ) in function of the target node fraction f for the random selection scheme. ( c ) For SF networks with ‹ k ›=5.6 and exponent γ =2.4, we show the normalized fraction of driver nodes ( α D ) as a function of the target node fraction f for the random scheme. ( d – f ) Local selection scheme. ( d ) The selection of an f =1/3 target node with the local scheme. ( e ) For ER networks with the same average degree as in b , we show the normalized fraction of driver nodes ( α D ) in function of the target node fraction f for the local scheme. ( f ) For SF networks with the same ‹ k › and γ as in c , we show the normalized fraction of driver nodes ( α D ) as a function of the target node fraction f for the local scheme. The black line describes the neutral case, that is, α D = f (or P D = fN D ) when the target control has the same efficiency as the full control. In each figure, we denote UB as the upper bound, GA as the greedy algorithm and LB as the lower bound of the minimum number of driver nodes to control an f fraction of target nodes. For ER networks, random target control is always less efficient than the full control, and for local target control efficiency depends on f . For SF networks random target control is as efficient as full control, but significant gains in efficiency are observed for local target control. Furthermore, for ER and SF networks local target control is more efficient than random target control. All results are averaged over 200 independent realizations of the networks with 10 4 nodes. Full size image In general, we find that the local target control scheme requires fewer driver nodes when compared with the random target control scheme. This can be explained as follows. The GA helps us obtain an approximately minimal set of driver nodes sufficient to control the target nodes. Yet, the size of the controllable subsystem (or equivalently, the dimension of the controllable subspace) can be larger than the size of the target node set. In other words, we may actually be able to control a larger subsystem than necessary. In Supplementary Fig. 3 , we show that the random target control scheme has larger controllable subsystems than the local target control scheme. This is true for any fraction f of target nodes. Hence the local control scheme is more efficient than the random control scheme. Furthermore, we find that α D is robust to changes in network size as shown in Supplementary Fig. 6 . Finally, since the hubs play an important role in complex networks, we study the case of controlling an f fraction of the highest in- and out-degree nodes as target nodes ( Supplementary Fig. 5 ). In general, we find that controlling the high-degree nodes reduces the minimum number of driver nodes. Target control efficiency The above observations raise a fundamental question: what kind of network topology is more efficient for target control and which control scheme (random or local) facilitates target control for a general f fraction of target nodes? To address this question, we define the overall target control efficiency in the Methods. The overall target control efficiency of two model networks (ER and SF) are shown in Fig. 5 as provided by simulations. When ‹ k ›=0 (a network with N isolated nodes), we have . That is, if we wish to control an f fraction of nodes we need to drive the same fraction of driver nodes as in the case of full control. We observe a peak of target control efficiency for SF networks with degree exponent γ ε[2, 3], which is the range of γ relevant for many real-world networks [37] , [38] ( Fig. 5a,c ). 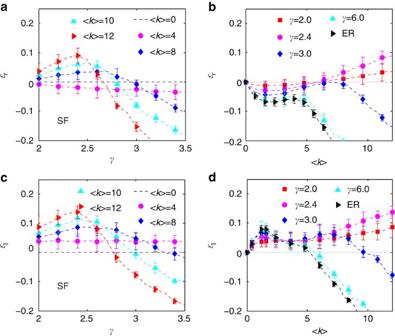Figure 5: Overall target control efficiency of model networks. (a,b) Random selection scheme. (a) The overall target control efficiency(equation (4)) for SF networks in function of degree exponentγfor different values of average degree ‹k› in the random scheme. (b) The overall target control efficiency(equation (4)) in function of the average degree ‹k› for different values of the degree exponentγfor SF networks and ER networks for random scheme. (c,d) Local selection scheme. (c) The overall target control efficiency(equation (4)) for SF networks in function of degree exponentγfor different values of average degree ‹k› for local scheme. (d) The overall target control efficiency(equation (4)) in function of the average degree ‹k› for different values of degree exponentγof SF networks and ER networks for local scheme. Fromaandbwe can see that for large ‹k› whenγis small the system has positive target control efficiency, but whenγis greater than a certain value, the efficiency decreases monotonically withγbecoming negative. Comparinga,bwith (c,d), we find that the local control can enhance the target control efficiency. The results are obtained by averaging over 200 realizations of networks with 104nodes. Figure 5: Overall target control efficiency of model networks. ( a , b ) Random selection scheme. ( a ) The overall target control efficiency (equation (4)) for SF networks in function of degree exponent γ for different values of average degree ‹ k › in the random scheme. ( b ) The overall target control efficiency (equation (4)) in function of the average degree ‹ k › for different values of the degree exponent γ for SF networks and ER networks for random scheme. ( c , d ) Local selection scheme. ( c ) The overall target control efficiency (equation (4)) for SF networks in function of degree exponent γ for different values of average degree ‹ k › for local scheme. ( d ) The overall target control efficiency (equation (4)) in function of the average degree ‹ k › for different values of degree exponent γ of SF networks and ER networks for local scheme. From a and b we can see that for large ‹ k › when γ is small the system has positive target control efficiency, but when γ is greater than a certain value, the efficiency decreases monotonically with γ becoming negative. Comparing a , b with ( c , d ), we find that the local control can enhance the target control efficiency. The results are obtained by averaging over 200 realizations of networks with 10 4 nodes. Full size image This optimal target control efficiency is likely due to the presence of the hubs. Indeed, starting from an ER network, we can fix the number of links and rewire the network to increase the degree of a preselected node, turning it into a hub. We find that the target control efficiency increases as we develop a hub ( Supplementary Fig. 4 ; Supplementary Note 4 ), explaining the increase of efficiency as we lower γ from γ >3 to γ ≈2.5. Overall, Fig. 5a suggests that many real-world networks may have been optimized for efficient target controllability. Interestingly, we find that networks, which are easier to control if we wish to achieve full control, that is, those with large average degree ‹ k › or large degree exponent γ [12] , do not show high efficiency for target control. Moreover, SF networks with 2≤ γ ≤3, which are harder to fully control than ER networks, have high random target control efficiency ( Fig. 5c ). Compared with ER networks, a SF network has lower local target control efficiency when the average degree ‹ k › is small but higher local target control efficiency when the average degree ‹ k › is large ( Fig. 5d ). Figure 5d also indicates the existence of a critical ‹ k › c so that when ‹ k ›>‹ k › c SF networks are more efficient than ER networks for target control. In general, sparse and homogeneous networks display high efficiency for target control, especially in the local scheme. Target control of real networks Next we apply the tools developed above to several real networks divided into seven categories, which are chosen for their diversity in applications and scope ( Fig. 6 ; Table 1 ). We find that networks from the same category display similar target control efficiency ( Fig. 6a,d ). Interestingly, only networks with large average degree (‹ k ›>‹ k › c >2.4) are more efficient than their randomized counterparts with respect to the local target control scheme, that is, (with values indicated in italics in Table 1 , column ‹ k › and in Fig. 6f ). This is in agreement with simulations ( Fig. 5d ). We observe that local target control markedly increases the control efficiency of neuronal networks ( Fig. 6e ). The opposite result is obtained for the power grid, finding that random target control is more efficient than the local control ( Fig. 6b,e ). This implies that the structure of the power grid is not optimized to facilitate local target control. For all gene networks target control efficiency is close to 0, indicating that they have evolved towards a topology that has comparable control efficiency within any sub-segment. Also, in the random target control scheme, the comparison between real networks and randomized networks support our earlier conclusion: real networks are optimized to have high random target control efficiency, because for almost all of them. The two counter-examples are the trust networks, which are extremely small, however, with only 32 and 67 nodes. The target control efficiency of real networks is summarized in Table 1 . 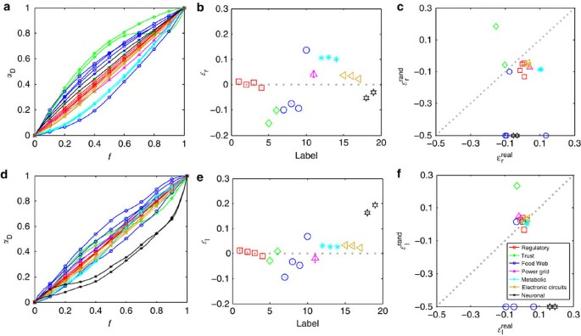Figure 6: Target control of real-world networks. (a–c) show random selection scheme. (a) The normalized fraction of driver nodes (αD) in function of the target node fractionffor the random scheme for 19 different real-world networks. Network labels are inTable 1. (b) The overall target control efficiency(equation (4)) of the real-world networks for the random scheme. (c) Comparing the target control efficiency of real networks with their randomized counterparts for the random scheme after, we randomly rewire each network using degree-preserving randomization. (d–f) Local selection scheme. (d) The normalized fraction of driver nodes (αD) in function of the target node fractionffor the local scheme for different real-world networks. (e) The overall target control efficiency(equation (4)) of real-world networks for the local scheme. (f) Comparing the target control efficiency of real networks with their randomized counterparts for the local scheme after, we randomly rewire each network using degree-preserving randomization. The results are averaged over 500 realizations. In general, real networks and more efficient than their randomized counterparts with respect to random target control. Figure 6: Target control of real-world networks. ( a – c ) show random selection scheme. ( a ) The normalized fraction of driver nodes ( α D ) in function of the target node fraction f for the random scheme for 19 different real-world networks. Network labels are in Table 1 . ( b ) The overall target control efficiency (equation (4)) of the real-world networks for the random scheme. ( c ) Comparing the target control efficiency of real networks with their randomized counterparts for the random scheme after, we randomly rewire each network using degree-preserving randomization. ( d – f ) Local selection scheme. ( d ) The normalized fraction of driver nodes ( α D ) in function of the target node fraction f for the local scheme for different real-world networks. ( e ) The overall target control efficiency (equation (4)) of real-world networks for the local scheme. ( f ) Comparing the target control efficiency of real networks with their randomized counterparts for the local scheme after, we randomly rewire each network using degree-preserving randomization. The results are averaged over 500 realizations. In general, real networks and more efficient than their randomized counterparts with respect to random target control. Full size image Table 1 The properties of the real network analysed in this paper. Full size table In this work, we studied the target controllability of complex networks. We developed a new theoretical approach, the k -walk theory, to identify the controllable sub-graph that one node can control, and a GA to identify an approximately minimum set of driver nodes to control a specified target set of nodes. We studied both random and local target control schemes and analysed how the network topology impacts the target control efficiency. The GA proposed in this work is efficient in finding the driver nodes for target control when the network structure is completely known. In reality, we have very incomplete maps of many real-world networks and the full controllability of networks with missing links has been recently addressed in ref. 39 . Note that if we add the missing links back, they will only enhance the target controllability of the system, unless the link weights satisfy some particular algebraic constraints, which is a typical zero-measure event. Our results raise several open questions: what higher-order network characteristics (such as communities, degree correlations) determine target controllability and target control efficiency? How to design the control inputs to steer the target nodes towards a desired final state? How to apply the GA to the study the target control of link dynamics? Finally, as discussed in the Methods section, our formulation considers the canonical linear time-invariant dynamics of a system. Extending these findings to networks with fully nonlinear dynamics may require connecting our current work with complimentary approaches that consider the basins of attraction that describe the steady-state properties of nonlinear dynamics [10] , [40] . Understanding these questions can significantly improve our understanding of the control principles of complex systems. Greedy algorithm The GA we introduce here is based, in part, on iterating the procedure for the lower-bound calculation to ultimately approximate the minimum set of driver nodes ( ) for target control ( Fig. 2d,e ). The lower-bound of P D can be calculated as follows: (1) Construct a bipartite graph , where the right side consists of all the target nodes, and the left side consists of all the nodes that can reach the target nodes. There is a link between node and if there is a link in the original directed network . (2) Find a maximum matching in . The number of unmatched nodes in yields the lower-bound of P D . The greedy algorithm works as follows. (1) Initialize the set to be the set of the unmatched nodes found from the lower-bound calculation. (2) Identify the set of nodes in that match the nodes in , and let this node set to be the new set and get a new bipartite graph. (3) Calculate a maximum matching in the updated bipartite graph and add unmatched nodes in to the set . (4) Repeat (2) and (3) until all nodes have been matched or are in the set . In Fig. 2d,e , we offer a specific example and the details of the GA. The proof of its sufficiency for target controllability is provided in Supplementary Fig. 2 and Supplementary Note 2 . Figure 2e can also be obtained by the k -walk theory, because the length of the path from the node 1 to each target node {1, 2, 4, 6, 7} is unique. Note that if the GA converges after only one iteration, we obtain the exact number for the minimum number of driver nodes for target control. A direct illustration of our algorithm’s utility is illustrated in Fig. 3 , where we consider control of the network shown in Fig. 2 . To control the entire network, we need at least three driver nodes. Indeed, as we show in Fig. 3a,b using these three nodes we can move the state of all nodes to the desired final state x i =10. But if we just want to control a subsystem {1, 2, 4, 6, 7} (highlighted in red in Fig. 2e ), the GA predicts that we need a single driver node, node 1. Indeed, as we show in Fig. 3c,d we can now move the state of the target nodes to the desired final state through an input to node 1 only. The nodes outside of the target list take arbitrary values as we do not control them. Target control efficiency We define the overall target control efficiency of an arbitrary network as denoting the efficiency of random and local target control scheme by and , respectively. For example, for the overall network efficiency is neutral, that is, to control an f fraction of target nodes we need fN D driver nodes. When , the network is less (or more) efficient than neutral expectation. Furthermore, , so corresponds to the most efficient case and shows the least efficient case. One example of the least efficient case is when only one driver node is needed to control the whole network. If we control any fraction of nodes, we still need one driver node, thus (observed for Food Web and Neuronal networks in Table 1 ). Note that target controllability for a specific fraction, α D ( f ), depends on the fraction f of driver nodes, but overall target control efficiency, , is a property of the whole network, independent of the fraction of target nodes. How to cite this article: Gao, J. et al. Target control of complex networks. Nat. Commun. 5:5415 doi: 10.1038/ncomms6415 (2014).